Advanced zinc-air batteries based on high-performance hybrid electrocatalysts Primary and rechargeable Zn-air batteries could be ideal energy storage devices with high energy and power density, high safety and economic viability. Active and durable electrocatalysts on the cathode side are required to catalyse oxygen reduction reaction during discharge and oxygen evolution reaction during charge for rechargeable batteries. Here we developed advanced primary and rechargeable Zn-air batteries with novel CoO/carbon nanotube hybrid oxygen reduction catalyst and Ni-Fe-layered double hydroxide oxygen evolution catalyst for the cathode. These catalysts exhibited higher catalytic activity and durability in concentrated alkaline electrolytes than precious metal Pt and Ir catalysts. The resulting primary Zn-air battery showed high discharge peak power density ~265 mW cm −2 , current density ~200 mA cm −2 at 1 V and energy density >700 Wh kg −1 . Rechargeable Zn-air batteries in a tri-electrode configuration exhibited an unprecedented small charge–discharge voltage polarization of ~0.70 V at 20 mA cm −2 , high reversibility and stability over long charge and discharge cycles. There is an urgent need for the development of efficient, safe and affordable energy storage devices for portable electronics, electrical vehicles and stationary grid storage [1] , [2] . In recent years, rechargeable metal-air batteries have attracted renewed interest as a possible energy storage solution. With ample supply of oxygen from the atmosphere, metal-air batteries have drastically higher theoretical energy density than traditional aqueous batteries and lithium ion batteries [3] , [4] , [5] . Zn-air batteries have been suggested to be a promising metal-air system for practical use [6] ( http://www.meridian-int-res.com/Projects/The_Zinc_Air_Solution.pdf retrieved on Oct 2012). Zn is the fourth most abundant metal in the earth’s crust, and could sustain large battery production to meet the growing demand of the global electrical vehicle industry ( http://www.meridian-int-res.com/Projects/The_Zinc_Air_Solution.pdf retrieved on Oct 2012). Primary Zn-air batteries have a high theoretical energy density about three times higher than the lithium ion technology [7] , and have been used in medical and telecommunication applications, such as miniature hearing aids and wireless messaging devices [7] . Nevertheless, the development of electrically rechargeable Zn-air batteries has been hampered by the lack of efficient, robust air catalysts as well as Zn anodes with high cyclability [5] , [6] , [7] . Here we demonstrate primary and rechargeable Zn-air batteries using highly active and durable air electrocatalysts based on high-performance non-precious metal oxide or hydroxide for oxygen reduction reaction (ORR) and/or oxygen evolution reaction (OER). Recently, we developed CoO and carbon nanotube (CNT) hybrid material as an ORR electrocatalyst with higher activity than standard 20 wt% Pt on Vulcan carbon black [8] , and Ni-Fe-layered double hydroxide (NiFe LDH) and CNT hybrid material as an OER electrocatalyst with activity and durability superior to 20 wt% Ir supported on Vulcan carbon black ( http://arxiv.org/abs/1303.3308 ). Carbon-free NiFe LDH was found to be a highly OER-active phase in alkaline solutions even without the need of hybridizing with CNTs ( http://arxiv.org/abs/1303.3308 ). The electrocatalytic performances of these catalysts are due to the novel phases of the inorganic nanoparticles, and the intimate bonding and electrical wiring to the underlying CNT networks further improve the catalyst activity. Using these electrocatalysts for the air cathode, we develop primary and rechargeable Zn-air batteries with significantly reduced ORR and OER overpotentials, and thus a high discharge power density of ~265 mW cm −2 , and a large energy density of >700 Wh kg −1 . Moreover, the high durability of the catalysts also leads to advanced rechargeable Zn-air batteries with long cycle life and high energy efficiency when operated in a tri-electrode configuration. Synthesis of air electrocatalysts The synthesis of ORR and OER hybrid electrocatalysts followed the general synthetic strategy developed in our lab [8] , [9] , [10] , [11] , [12] , [13] . In brief, transition metal salts and mildly oxidized multi-walled CNTs were dispersed in selected solvents. Controlled hydrolysis of metal precursors at a low temperature led to the selective nucleation, growth of metal oxide and hydroxide nanostructures on CNTs, which were further subjected to solvothermal reactions or gas-phase annealing in ammonia environment at elevated temperatures to afford the desired phase, crystallinity of metal oxide or hydroxide and the reduction of oxidized CNTs with N-doping (see Methods). Through careful selections of precursors, solvents, reaction temperatures and gas environments, we obtained uniform-sized CoO nanocrystals on N-doped CNTs (CoO/N-CNT, Fig. 1a–c ) and NiFe LDH ultrathin nanoplates on multi-walled CNTs (NiFe LDH/CNT, with a nominal Ni:Fe=5, Fig. 1d–f ). Carbon-free NiFe LDH nanoplates were also synthesized without the addition of CNTs. The composition and phase of the materials were characterized and analysed in detail [8] ( http://arxiv.org/abs/1303.3308 ). 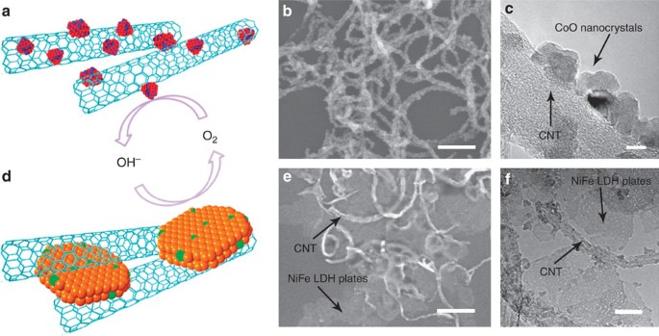Figure 1: ORR and OER electrocatalysis. Strongly coupled inorganic/CNT hybrids for ORR and OER electrocatalysis with low overpotentials. (a–c) Schematic structure, scanning electron microscopy (SEM) and transmission electron microscopy (TEM) images of CoO/N-CNT hybrid. (d–f) Schematic structure, SEM and TEM images of NiFe LDH/CNT hybrid. Scale bars are 200 nm, 5 nm, 200 nm and 20 nm, respectively, inb,c,eandf. Figure 1: ORR and OER electrocatalysis. Strongly coupled inorganic/CNT hybrids for ORR and OER electrocatalysis with low overpotentials. ( a – c ) Schematic structure, scanning electron microscopy (SEM) and transmission electron microscopy (TEM) images of CoO/N-CNT hybrid. ( d–f ) Schematic structure, SEM and TEM images of NiFe LDH/CNT hybrid. Scale bars are 200 nm, 5 nm, 200 nm and 20 nm, respectively, in b , c , e and f . Full size image Activity and durability of hybrid electrocatalysts for ORR and OER We evaluated the electrocatalytic ORR and OER performance of CoO/N-CNT and NiFe LDH/CNT in 6 M KOH using a standard three-electrode system with a Hg/HgO reference electrode ( Supplementary Fig. S1 ). Catalyst powders were dispersed in a Nafion ethanol solution with a Nafion-to-catalyst mass ratio of 0.1 to form a homogeneous catalyst ink aided by ultrasonication, and then uniformly drop-casted onto a Teflon-treated carbon fibre paper electrode (or gas diffusion layer) to achieve a catalyst loading of 1 mg cm −2 (see Methods). The use of hydrophobic carbon fibre paper as the air electrode was critical to ORR, as it provided a highly developed three-phase boundary for the electrocatalytic reduction of oxygen [9] . For comparison, commercial 20 wt% Pt and 20 wt% Ir supported on Vulcan carbon black (from Premetek Co.) were measured as the ORR and OER benchmarks, respectively ( Fig. 2a ). On the cathodic branch, CoO/N-CNT exhibited an ORR onset potential ~20 mV negative to that of Pt/C, but its activity quickly caught up and surpassed the latter at current densities relevant to Zn-air battery operation. At a cathodic current density of 100 mA cm −2 , the CoO/N-CNT catalyst operated at >20 mV more positive potential than Pt/C. Among all Co- or Mn-based ORR hybrid catalysts developed in our group [8] , [9] , [10] , [11] , CoO/N-CNT showed the highest ORR electrocatalytic activity and outperformed the Pt/C benchmark in alkaline solutions. The CoO/N-CNT was also active for OER in the anodic potential regime, making it an appealing bi-functional catalyst in alkaline solutions. However, we found that the OER activity of the catalyst was surpassed by the NiFe LDH/CNT hybrid and carbon-free NiFe LDH nanoplates ( http://arxiv.org/abs/1303.3308 ). At an anodic current density of 50 mA cm −2 , the polarization curve of NiFe LDH/CNT was ~20 mV more negative than the Ir/C benchmark, and ~40 mV more negative than CoO/N-CNT ( Fig. 2a ). 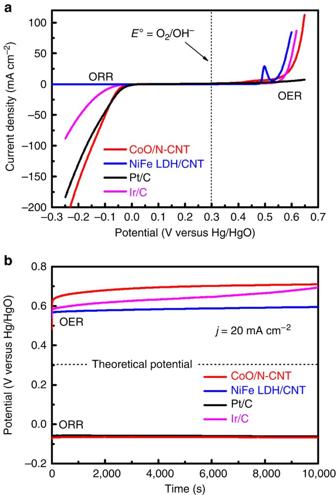Figure 2: High-performance electrocatalysts based on inorganic/CNT hybrid materials over precious metals. (a) ORR and OER polarization curves and (b) chronopotentiometry (i~t) measurements of CoO/N-CNT and NiFe LDH/CNT compared with 20 wt% Pt/C and 20 wt% Ir/C benchmarks in 6 M KOH on Teflon-coated carbon fibre paper (CFP) electrodes. The catalyst loading on CFP electrodes was 1 mg cm−2for all materials. The anodic peak of FeNi LDH/CNT in (a) is due to the oxidation from Ni2+to Ni3+or Ni4+in α-phase Ni(OH)2before OER24. Figure 2: High-performance electrocatalysts based on inorganic/CNT hybrid materials over precious metals. ( a ) ORR and OER polarization curves and ( b ) chronopotentiometry ( i ~ t ) measurements of CoO/N-CNT and NiFe LDH/CNT compared with 20 wt% Pt/C and 20 wt% Ir/C benchmarks in 6 M KOH on Teflon-coated carbon fibre paper (CFP) electrodes. The catalyst loading on CFP electrodes was 1 mg cm −2 for all materials. The anodic peak of FeNi LDH/CNT in ( a ) is due to the oxidation from Ni 2+ to Ni 3+ or Ni 4+ in α-phase Ni(OH) 2 before OER [24] . Full size image Other than high ORR and OER activity, the durability of electrocatalysts is another important parameter, as it determines the cycle life of metal-air batteries. Chronopotentiometry ( i ~ t ) measurements were carried out at a constant cathodic or anodic current density of 20 mA cm −2 ( Fig. 2b ). Both CoO/N-CNT and Pt/C exhibited high ORR stability with no significant activity loss over ~3 h, whereas the OER catalysts suffered activity loss to different extents as manifested by their gradually increasing working potential over time. Among them, NiFe LDH/CNT was the most durable OER catalyst with an overpotential increase of ~30 mV during the course of experiment, in sharp contrast to Ir/C that showed >100 mV overpotential increase. While the instability of Ir catalysts in alkaline electrolytes was well documented [14] , the OER activity decay of NiFe LDH/CNT was much slower and likely related to structural transformation of the NiFe LDH phase. The high ORR and OER activity and durability of these hybrid electrocatalysts were attributed to the strong coupling effect between nanoscale inorganic particles and conducting CNT substrate [8] , [12] , [13] ( http://arxiv.org/abs/1303.3308 ). Importantly we found that carbon-free NiFe LDH nanoplates alone were highly OER active in alkaline solutions, more so than previous Ni- and Fe-based compounds due to the novel LDH phase and material morphology (ultrathin nanoplates with ~10 atomic layers) ( http://arxiv.org/abs/1303.3308 ). Primary Zn-air batteries To construct primary Zn-air batteries, we used the CoO/N-CNT ORR electrocatalyst loaded on the carbon fibre paper electrode as the air cathode and paired it with a Zn foil in 6 M KOH ( Fig. 3a ). The battery had an open circuit voltage of ~1.40 V. At a voltage of 1.0 V, it showed a high current density of ~200 mA cm −2 . The peak power density was 265 mW cm −2 reached at 0.70 V ( Fig. 3b ). Both the current density at 1 V and peak power density were significantly improved over previous reports on Zn-air primary batteries ( Supplementary Table S1 , >30% gain in current density and ~15 % gain in power density over previous batteries) [15] , [16] , [17] , [18] , and slightly outperformed the battery made with Pt/C ORR catalyst at the same mass loading ( Fig. 3b ) as the result of the higher ORR activity of CoO/N-CNT. 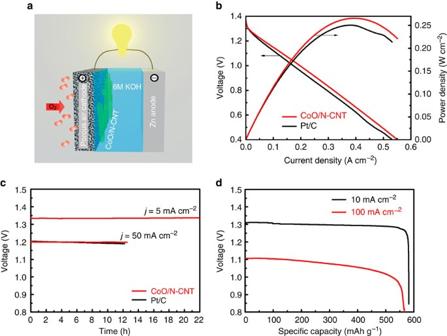Figure 3: Primary Zn-air battery with CoO/N-CNT ORR catalyst as the cathode. (a) A schematic of the primary Zn-air battery. (b) A polarization curve (V~i) and corresponding power density plot of the battery using CoO/N-CNT as the cathode catalyst compared with the battery using commercial Pt/C catalyst. (c) Long-time discharge curve of a primary batteries using CoO/N-CNT cathode catalyst at two different current densities compared with the battery using Pt/C as the cathode catalyst. (d) Typical discharge curves of primary Zn-air batteries with CoO/N-CNT as the cathode catalyst under continuous discharge until complete consumption of Zn at two different current densities. Specific capacity was normalized to the mass of consumed Zn. Figure 3: Primary Zn-air battery with CoO/N-CNT ORR catalyst as the cathode. ( a ) A schematic of the primary Zn-air battery. ( b ) A polarization curve ( V ~ i ) and corresponding power density plot of the battery using CoO/N-CNT as the cathode catalyst compared with the battery using commercial Pt/C catalyst. ( c ) Long-time discharge curve of a primary batteries using CoO/N-CNT cathode catalyst at two different current densities compared with the battery using Pt/C as the cathode catalyst. ( d ) Typical discharge curves of primary Zn-air batteries with CoO/N-CNT as the cathode catalyst under continuous discharge until complete consumption of Zn at two different current densities. Specific capacity was normalized to the mass of consumed Zn. Full size image Primary Zn-air batteries made with CoO/N-CNT catalyst were very robust. When galvanostatically discharged at 5 mA cm −2 for ~22 h or at 50 mA cm −2 for ~12 h, no obvious voltage drop was observed ( Fig. 3c ) owing to the stability of CoO/N-CNT for ORR [8] . As discharge continued, the Zn foil was gradually thinned, and the electrolyte accumulated more and more soluble zinc salts. The battery eventually ceased functioning when all the Zn metal was consumed ( Fig. 3d ). The specific capacity normalized to the mass of consumed Zn was ~570 mAh g −1 , corresponding to a high energy density >700 Wh kg −1 . Interestingly, we found that simply replenishing the metal anode and electrolyte could regenerate the battery for subsequent runs at the same performance level with the same CoO/N-CNT cathode, again suggesting the durability of hybrid electrocatalyst. Recently, Zn-air fuel cells or Zn-air flow batteries have been proposed and demonstrated to power electric vehicles with high power, long driving distance and commercial viability [19] , [20] ( http://www.electric-fuel.com/evtech/ef-tech-brochure.pdf , retrieved Oct 2012). They can be quickly refuelled with fresh metallic Zn powders, and the produced zincate species in the electrolyte can be collected and recovered in off-site regeneration facilities ( http://www.electric-fuel.com/evtech/ef-tech-brochure.pdf , retrieved Oct 2012). Our CoO/N-CNT ORR catalyst is ideally suited for such refuelling primary Zn-air batteries owing to the exceptional ORR activity and durability. Rechargeable Zn-air batteries For rechargeable Zn-air batteries, we investigated the combination of CoO/N-CNT and NiFe LDH/CNT as air catalysts. First, we mixed these materials and loaded them onto a single cathode for charge and discharge cycling experiments ( Fig. 4a ). The electrolyte used was 6 M KOH with 0.2 M zinc acetate (dissolved in KOH to form zincate, Zn(OH) 4 2− ) to ensure reversible Zn electrochemical reactions at the anode [21] . Such a battery exhibited cycling stability when charged and discharged galvostatically at low current densities (5–10 mA cm −2 ) in short cycle times (200–2,000 s per charge or discharge period) ( Fig. 4b ). However, the battery discharge performance deteriorated noticeably at higher current densities and through long cycle times (for example, 20 mA cm −2 , 20 h per cycle; Fig. 4c ). The discharge overpotential needed for the second cycle was 200–250 mV larger than the first cycle. We found that this was owing to ORR electrocatalytic activity loss caused by the first charging step, during which the oxidation of CoO/N-CNT occurred to a certain extent. 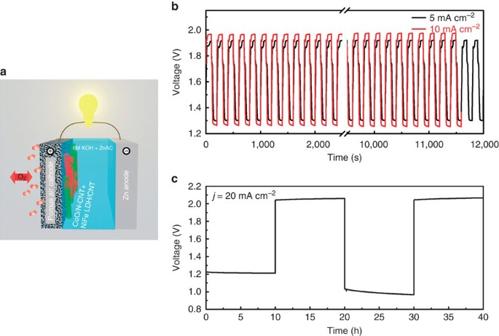Figure 4: Rechargeable Zn-air batteries with hybrid catalysts as the cathode. CoO/N-CNT ORR and FeNi LDH/CNT OER hybrid catalysts are mixed in a single cathode. (a) A schematic structure of the battery. (b) Cycling data at 5 and 10 mA cm−2, respectively, in short cycle periods (200 s per cycle). (c) Cycling data at 20 mA cm−2in long cycle periods (20 h per cycle). Figure 4: Rechargeable Zn-air batteries with hybrid catalysts as the cathode. CoO/N-CNT ORR and FeNi LDH/CNT OER hybrid catalysts are mixed in a single cathode. ( a ) A schematic structure of the battery. ( b ) Cycling data at 5 and 10 mA cm −2 , respectively, in short cycle periods (200 s per cycle). ( c ) Cycling data at 20 mA cm −2 in long cycle periods (20 h per cycle). Full size image Oxidation under the positive potentials needed for OER caused the loss of strong coupling between CoO and CNTs. Transmission electron microscopy image of the CoO/N-CNT after ORR–OER cycling showed detachment of metal oxide nanocrystals from CNT supports accompanied by aggregation ( Supplementary Fig. S3 ). This result suggested that even though the CoO/N-CNT hybrid exhibited excellent stability for ORR within negative potential regimes, oxidative potentials during charging of Zn-air batteries could cause ORR activity decay due to the loss of strong CoO-carbon coupling that was responsible for the high ORR activity of the hybrid in the first place [9] . To circumvent the deactivation problem of ORR catalyst upon exposure to OER potential regimes, we explored rechargeable Zn-air batteries in a tri-electrode configuration [6] . As shown in Fig. 5a , OER and ORR electrocatalysts were loaded onto two separate electrodes for charge and discharge, respectively. ORR electrode connected to the Zn anode only for discharge, thus avoiding exposure to positive potentials. In this configuration, these two electrocatalysts were decoupled and could be optimized individually. Also, we found that highly conducting and porous Ni foam was a much better current collector than carbon fibre paper for OER electrocatalysis. We found that a high loading of carbon-free FeNi LDH nanoplates on the Ni foam (5 mg cm −2 ) afforded an OER electrode with optimal activity and stability. Even though the OER activity was 30–40 mV worse than FeNi LDH/CNT hybrid or Ir/C on Ni foam at the same mass loading, its durability were improved with only 20 mV overpotential increase over 100 h of operation when anodically biased at 20 mA cm −2 ( http://arxiv.org/abs/1303.3308 ). 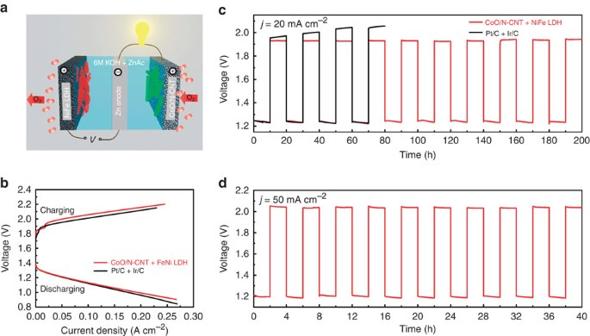Figure 5: Rechargeable Zn-air batteries in a tri-electrode configuration. (a) A schematic of the tri-electrode configuration with CoO/N-CNT ORR catalyst loaded on CFP electrode (1 mg cm−2) and carbon-free NiFe LDH OER catalyst loaded on Ni foam (~5 mg cm−2) electrode for discharge and charge, respectively. (b) Charge and discharge polarization (V~i) curves of the tri-electrode Zn-air battery using CoO/N-CNT and NiFe LDH (red) compared with the one using Pt/C and Ir/C (black). (c) Cycling performance of the tri-electrode Zn-air battery using CoO/N-CNT and NiFe LDH at 20 mA cm−2and a 20-h cycle period compared with the tri-electrode battery using Pt/C and Ir/C. (d) The same CoO/N-CNT and NiFe LDH electrodes fromcwere used for a subsequent cycling experiment with a fresh Zn anode at 50 mA cm−2and a 4-h cycle period. Figure 5: Rechargeable Zn-air batteries in a tri-electrode configuration. ( a ) A schematic of the tri-electrode configuration with CoO/N-CNT ORR catalyst loaded on CFP electrode (1 mg cm −2 ) and carbon-free NiFe LDH OER catalyst loaded on Ni foam (~5 mg cm −2 ) electrode for discharge and charge, respectively. ( b ) Charge and discharge polarization ( V ~ i ) curves of the tri-electrode Zn-air battery using CoO/N-CNT and NiFe LDH (red) compared with the one using Pt/C and Ir/C (black). ( c ) Cycling performance of the tri-electrode Zn-air battery using CoO/N-CNT and NiFe LDH at 20 mA cm −2 and a 20-h cycle period compared with the tri-electrode battery using Pt/C and Ir/C. ( d ) The same CoO/N-CNT and NiFe LDH electrodes from c were used for a subsequent cycling experiment with a fresh Zn anode at 50 mA cm −2 and a 4-h cycle period. Full size image Figure 5b shows the charge and discharge polarization curves of a rechargeable Zn-air battery in the tri-electrode configuration using NiFe LDH loaded on Ni foam for OER electrode and CoO/N-CNT on carbon fibre paper for ORR electrode. The battery exhibited similar current densities as the rechargeable battery made with 20 wt% Pt/C and 20 wt% Ir/C as the ORR and OER electrodes, respectively, at the same charging or discharging voltage. The charge–discharge voltage gap at 20 mA cm −2 was ~0.70 V (voltage polarization contributed by the sum of OER and ORR overpotentials at the air electrodes, see Supplementary Fig. S4 ), much smaller than previous reports by up to ~0.8 V ( Supplementary Table S2 ) [22] , [23] . Importantly, when repeatedly charged or discharged at 20 mA cm −2 for a total of 200 h with a 20 h per cycle period, the battery showed high cycling stability, much improved over rechargeable batteries in the single cathode configuration in which ORR and OER catalysts were mixed together ( Fig. 5c versus Fig. 4c ). Furthermore, the same ORR and OER electrodes were used for subsequent cycling experiments with a fresh Zn anode at 50 mA cm −2 for additional 40 h with a 4 h per cycle period ( Fig. 5d ). Again no significant voltage change can be discerned on both the charge and discharge segments. After these rigorous measurements, the electrocatalysts still exhibited no obvious degradation, without setting a limit to ORR and OER operations for long cycling times of Zn-air batteries. The calculated energy efficiency was ~65% at 20 mA cm −2 , and maintained ~60% at 50 mA cm −2 due to the excellent ORR and OER activity of the electrocatalysts. Even though the tri-electrode configuration inevitably increased the battery volume, the gain in cycling stability was certainly appealing and significant. Among a handful of reports on rechargeable Zn-air batteries ( Supplementary Table S2 ), few have reported the long-term cycling stability under long charge–discharge periods. One report was by Toussaint et al . [6] , in which a rechargeable battery was cycled in a similar tri-electrode configuration at 5–15 mA cm −2 for a total of 120 h with a 30-h cycle period. The reported cycling stability was good, but the battery had larger charge–discharge voltage polarization compared with our work (>0.9 versus 0.7 V), and lower energy efficiency (50% versus 65%). In our control experiment, rechargeable Zn-air batteries made with Pt/C and Ir/C combination in the tri-electrode configuration showed a stable discharge voltage but the charging voltage increased continuously (due to the gradual deactivation of IrO x in alkaline electrolytes), and became much less active in just four cycles ( Fig. 5c black curve). In summary, we investigate two novel electrocatalysts CoO/N-CNT hybrid and NiFe LDH for ORR and OER electrocatalysis in 6 M KOH for primary and rechargeable Zn-air batteries. The activity and durability of these materials outperformed precious metal electrocatalysts, and show promise as air catalysts in aqueous rechargeable metal-air batteries. We construct primary Zn-air batteries using the CoO/N-CNT hybrid ORR catalyst for the air cathode. The battery delivers large discharge current densities with an unprecedented peak power density of ~265 mW cm −2 . The robustness of our ORR hybrid catalyst allows the battery to run continuously and consistently by refuelling the Zn anode and electrolyte periodically, presenting an ideal air catalyst for Zn-air fuel cells or Zn-air flow batteries for electrical vehicles. However, we find that the catalytic activity of CoO/N-CNT hybrid ORR catalysts decreases when exposed to OER potential regimes. To bypass this problem, we devise rechargeable Zn-air batteries in the tri-electrode configuration with separate OER and ORR electrode for charge and discharge, respectively. The battery shows the smallest charge–discharge polarization of ~0.70 V and excellent cycling stability over repeated, 4- to 20-h-long charge–discharge cycles at 20–50 mA cm −2 . Thus, we succeed in advancing the air cathode catalysts for both primary and rechargeable Zn-air batteries. Rechargeable Zn-air batteries still face other challenges such as the dendritic growth of Zn metal on charging and CO 2 management, which should be addressed before practical rechargeable Zn-air batteries are made [5] , [6] , [21] . Materials synthesis The preparation of CoO/N-CNT and NiFe LDH/CNT followed previous reports [8] ( http://arxiv.org/abs/1303.3308 ). Briefly, multi-walled CNTs (FloTube 9000, CNano Technology Ltd.) was first purified to remove metal impurities, and mildly oxidized by modified Hummers’ method with a KMnO 4 -to-carbon weight ratio of 1. For CoO/N-CNT hybrid, 18 ml of oxidized CNTs was dispersed in 24 ml of ethanol and 0.5 ml water, to which 0.6 ml of 0.6 M Co(OCH 2 CH 3 ) 2 and 0.5 ml of 30 wt% NH 4 OH aqueous solution was added in sequence. The reaction was kept at 80 °C for 20 h under magnetic stirring. Resulting products were collected by centrifugation, washed and dried by lyophilization. They were further annealed at 400 °C for 2 h at 10% NH 3 /Ar atmosphere to afford the final product. For NiFe LDH/CNT, 6 mg of oxidized CNTs were dispersed in 12 ml of anhydrous N , N -dimethylformamide, to which 1.2 ml of 0.2 M Ni(OCH 2 CH 3 ) 2 and 0.24 ml of 0.2 M Fe(NO 3 ) 3 aqueous solution were added. The reaction was kept at 80 °C for 4 h under magnetic stirring. Resulting products were collected and re-dispersed in a mixture of 12 ml of N , N -dimethylformamide and 24 ml of water. They were then transferred to a Teflon-lined stainless steel autoclave for solvothermal reaction at 120 °C for 12 h, followed by another solvothermal treatment at 160 °C for 2 h. The final products were collected by centrifugation, washed and dried by lyophilized. Carbon-free NiFe LDH was synthesized without the addition of oxidized CNTs under otherwise identical conditions. Electrochemical measurements Four milligrams of hybrid catalysts were dispersed in 1 ml of ethanol and 8 μl of 5 wt% Nafion solution assisted by ultrasonication >30 min to form a homogeneous catalyst ink. Catalysts were uniformly loaded onto Teflon-treated carbon fibre paper (AvCarb P75T, Fuel Cell Store) to achieve a loading of 1 mg cm −2 . The electrochemical evaluations of individual catalysts (ORR and OER polarization curve and stability) were performed in a home-built three-electrode electrochemical cell using an Hg/HgO electrode (filled with 6 M KOH) as the reference, a graphite rod as the counter electrode and the carbon fibre paper electrode as the working electrode ( Supplementary Fig. S1 ). Before the start of each measurement, the 6 M KOH electrolyte was bubbled with O 2 for > 10 min. A flow of O 2 was maintained over the electrolyte during the measurement to ensure its continued O 2 saturation. Polarization data were collected using linear sweep voltammetry at a scan rate of 5 mV s −1 with automatic iR compensation. Chronopotentiometry ( i ~ t ) data were manually corrected for iR loss. For comparison, commercial 20 wt% Pt and 20 wt% Ir on Vulcan carbon black (Premetek Co.) were measured at the same condition. Primary and rechargeable Zn-air batteries were tested in home-built electrochemical cells ( Fig. 3a , Fig. 5a and Supplementary Fig. S2 ). For primary cells, a two-electrode configuration was used by pairing CoO/N-CNT loaded on a carbon paper electrode (1 cm 2 , catalyst loading 1 mg) with a Zn foil (Alfa Aesar) in 30–40 ml of 6 M KOH. For rechargeable Zn-air cells, a tri-electrode configuration was used with CoO/N-CNT loaded on a carbon paper electrode (1 cm 2 , catalyst loading 1 mg) for discharge, carbon-free NiFe LDH nanoplates loaded on a Ni foam (1 cm 2 , catalyst loading ~5 mg) for charge and a Zn foil anode in 30–40 ml of 6 M KOH with 0.2 M zinc acetate dissolved to form zincate. During battery measurements, oxygen (99.6% from Praxair) was continuously fed to the cathode. It was humidified by passing through a separate liquid water container before entering the cell. The battery internal impedance was measured to be 1.0~1.5 Ω at the open circuit condition. How to cite this article: Li, Y. et al . Advanced zinc-air batteries based on high-performance hybrid electrocatalysts. Nat. Commun. 4:1805 doi: 10.1038/ncomms2812 (2013).